Efficient hole-blocking layer-free planar halide perovskite thin-film solar cells Efficient lead halide perovskite solar cells use hole-blocking layers to help collection of photogenerated electrons and to achieve high open-circuit voltages. Here, we report the realization of efficient perovskite solar cells grown directly on fluorine-doped tin oxide-coated substrates without using any hole-blocking layers. With ultraviolet–ozone treatment of the substrates, a planar Au/hole-transporting material/CH 3 NH 3 PbI 3- x Cl x /substrate cell processed by a solution method has achieved a power conversion efficiency of over 14% and an open-circuit voltage of 1.06 V measured under reverse voltage scan. The open-circuit voltage is as high as that of our best reference cell with a TiO 2 hole-blocking layer. Besides ultraviolet–ozone treatment, we find that involving Cl in the synthesis is another key for realizing high open-circuit voltage perovskite solar cells without hole-blocking layers. Our results suggest that TiO 2 may not be the ultimate interfacial material for achieving high-performance perovskite solar cells. Organic–inorganic lead halide perovskite solar cells have attracted much attention in recent years. The power conversion efficiency (PCE) of lead halide perovskite-based solar cells has rapidly increased from 3.8 to ~20.1% (certified) in just 5 years [1] , [2] , [3] , [4] , [5] , [6] , [7] , [8] . Lead halide perovskite solar cells use either the mesoscopic or the planar cell architecture. Regardless of the cell architecture, high-efficiency lead halide perovskite solar cells exclusively use hole-blocking layers (HBLs)/electron-transporting layers (ETLs) and hole-transporting layers (HTLs)/electron-blocking layers (EBLs). These intrinsic interfacial layers are believed critically necessary for achieving high open-circuit voltages ( V OC ’s) and efficiencies because they promote effective carrier separations and charge recombination reduction at the front contacts, typically transparent conducting oxides such as fluorine-doped tin oxide (FTO) or indium-doped tin oxide-coated glass, and back contacts, typically metals such as Ag or Au. In the inverted structures, efficient perovskite solar cells have been achieved using organic HBLs and EBLs [9] . In the regular structures, the most used HBL/ETL and HTL/EBL materials reported in literature are TiO 2 and 2,2′,7,7′-tetrakis-( N , N -di-p-methoxyphenylamine)-9,9′-spirobifluorene (spiro-OMeTAD), respectively. A report has also shown that Y doping of TiO 2 ETL can improve the cell performance [6] . The reason why spiro-OMeTAD is a good HTL material for achieving high-efficiency cells has been investigated [10] . Recently, perovskite solar cells using poly(triaryl amine) HTLs have achieved the highest certified efficiency [7] . Significant efforts have been paid to search for alternative HBL and HTL materials or even to eliminate HTL layer [11] , [12] , [13] , [14] . Some lead halide perovskite solar cells without HTLs have achieved reasonable conversion efficiencies. It has been shown that the remnant PbI 2 layer in a CH 3 NH 3 PbI 3 film prepared by a two-step method can act as a HBL [15] . There are many oxides, for example, ZnO, In 2 O 3 and SnO 2 , that exhibit similar or even better electronic and optical properties than TiO 2 . Theoretically, these oxides should be as good HBL materials as TiO 2 . For example, perovskite solar cells using ZnO as HBL have achieved PCEs as high as 15.7%. To further understand the operation mechanism of lead halide perovskite solar cells and to further improve the cell performance, it is important to understand whether or not TiO 2 is the ultimate HBL for achieving high-efficiency cells in the regular structure. In this paper, we report on the realization of efficient planar lead halide perovskite solar cells grown directly on FTO substrates without any HBLs. By applying ultraviolet–ozone (UVO) treatment to the FTO substrates, a simple planar Au/spiro-OMeTAD/CH 3 NH 3 PbI 3- x Cl x /FTO cell processed by a low-temperature solution method has achieved a PCE of over 14% and a V OC of 1.06 V measured under the reverse voltage scan with a scan rate of 0.1 V s −1 . The V OC is as high as our best reference device using a TiO 2 HBL (PCE=16.07%, V OC =1.06 V) measured with the same voltage scan and rate. The perovskite absorbers were deposited by the one-step process and there are no obvious unreacted PbI 2 layers at FTO/perovskite interfaces to act as HBLs. Our results, therefore, strongly suggest that TiO 2 may not be an ultimate HBL material for achieving high-efficiency lead halide perovskite solar cells. We show that involving Cl in the synthesis process and applying UVO treatment to the FTO substrates are two key factors for achieving high V OC lead halide perovskite solar cells without any HBLs. The UVO treatment improves the perovskite film coverage, and, therefore, the fill factor (FF) and the V OC . Cl may segregate to and passivate FTO/CH 3 NH 3 PbI 3- x Cl x interfaces and, thus, improves the V OC . Our results reveal that alternative HBL materials or cell structures should be explored to further improve the performance of lead halide perovskite solar cells. 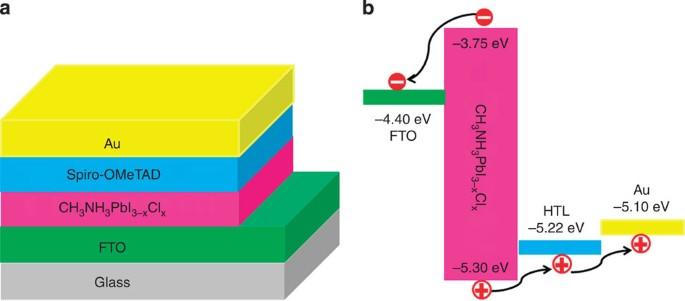Figure 1: Device architecture and energy diagram. (a) Schematic view of the perovskite solar cell configuration: Glass substrate, FTO front contact, CH3NH3PbI3-xClxfilm, spiro-OMeTAD HTL and Au back contact. (b) Energy band diagram of the FTO/CH3NH3PbI3-xClx/spiro-OMeTAD HTL/Au solar cell showing the separation and collection of photogenerated carriers. Device structure Figure 1a shows the device structure of our perovskite solar cells grown directly on FTO substrates without any HBLs. The perovskite films were directly coated on FTO substrates by a one-step spin-coating method. Following the deposition of the perovskite layer, a spiro-OMeTAD HTL (~250 nm) was deposited by spin coating. The cells were finished with thermally evaporated Au back contacts. The FTO substrates have a sheet resistance of 14 Ohms per square. Therefore, the FTO layers are the n ++ electrodes. Reports in literature have shown that some lead halide perovskite solar cells behave as p-i-n cells [3] , [16] , [17] , [18] . Our lead halide perovskites thin films are highly resistive and have low carrier concentrations, typically below the sensitivity of our Hall measurement system (~10 14 cm −3 ). Therefore, the operation mechanism for our cells may be similar to that of a p-i-n cell. Figure 1b shows the possible transportation of the photogenerated carriers and the energy band diagram of cells. The Au back contact makes good Ohmic contact to the p-type spiro-OMeTAD HTL ( Supplementary Fig. 1 ). Figure 1: Device architecture and energy diagram. ( a ) Schematic view of the perovskite solar cell configuration: Glass substrate, FTO front contact, CH 3 NH 3 PbI 3- x Cl x film, spiro-OMeTAD HTL and Au back contact. ( b ) Energy band diagram of the FTO/CH 3 NH 3 PbI 3- x Cl x /spiro-OMeTAD HTL/Au solar cell showing the separation and collection of photogenerated carriers. Full size image Because halide perovskite-based solar cells typically use very thin absorber layers (300–500 nm), it is critical to form perovskite thin films with full coverages and smooth surfaces. This is particularly important for the planar cell architecture because an incomplete coverage of a perovskite film results in low-resistance shunting paths and low light absorption in the solar cell. Significant efforts have been developed to improve film coverage and crystalline quality [19] , [20] , [21] . We found that the residual organic species or surface–OH basis group absorbed on the FTO substrates have detrimental effects on the formation of smooth perovskite thin films. These organic contaminants make the FTO substrates somewhat hydrophobic, thereby leading to a high contact angle for the polar solvents and a low wettability for the substrates. For spin-coating depositions, these effects result in rough perovskite thin films. Even after careful chemical cleaning, the surfaces of FTO substrates still contain chemisorbed small organic species. UVO or O 2 plasma treatment is widely used as a cleaning process [22] , [23] , [24] . We found that UVO treatment can effectively remove the residual organic species and, therefore, significantly reduce the contact angle of the polar solvents ( Supplementary Fig. 2 ). As a result, perovskite thin films with improved smoothness and coverage were obtained. 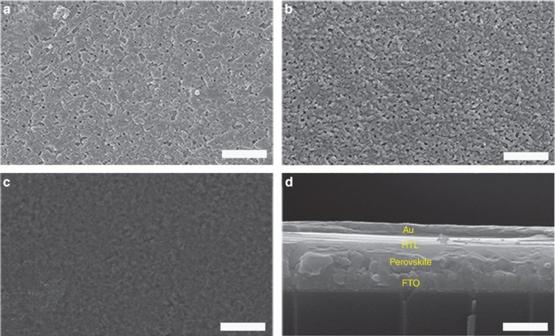Figure 2: Film and device morphologies. Top-view SEM images of the CH3NH3PbI3-xClxfilms on FTO (a) with and (b) without UVO treatment. Scale bar, 10 μm. (c) Top-view SEM image of the HTL on a CH3NH3PbI3-xClxfilm deposited on FTO with UVO treatment. Scale bar, 10 μm. (d) Cross-sectional SEM image of a complete device. Scale bar, 1 μm. Figure 2a,b shows secondary electron micrographs (SEMs) of CH 3 NH 3 PbI 3- x Cl x perovskite thin films grown on FTO substrates with and without UVO treatment, respectively. Based on device performance, the optimal UVO treatment time was found to be ~30 min. It is seen that the CH 3 NH 3 PbI 3- x Cl x perovskite thin films deposited on FTO substrates with UVO treatment exhibit larger grains and a lower density of pin holes than the films deposited on FTO substrates without UVO treatment. Because of the improved surface smoothness, the spiro-OMeTAD HTL can be coated smoothly, as shown in Fig. 2c . The cross-sectional SEM image of a planar perovskite-based solar cell grown directly on FTO-coated glass is shown in Fig. 2d , revealing no compact layer, mesoporous layer or porous scaffold supporting layer. For comparison, an SEM image taken from a CH 3 NH 3 PbI 3- x Cl x perovskite thin film deposited on a FTO substrate without UVO treatment is shown in Supplementary Fig. 3 . The perovskite film is less smooth as compared with the films deposited on UVO-treated FTO substrates. Figure 2: Film and device morphologies. Top-view SEM images of the CH 3 NH 3 PbI 3- x Cl x films on FTO ( a ) with and ( b ) without UVO treatment. Scale bar, 10 μm. ( c ) Top-view SEM image of the HTL on a CH 3 NH 3 PbI 3- x Cl x film deposited on FTO with UVO treatment. Scale bar, 10 μm. ( d ) Cross-sectional SEM image of a complete device. Scale bar, 1 μm. Full size image Lead halide perovskites exhibit extremely high optical absorption and high defect tolerance [25] , [26] . The spin-coated CH 3 NH 3 PbI 3- x Cl x perovskite thin films were examined by ultraviolet–visible spectroscopy, X-ray diffraction and room temperature photoluminescence (PL). The results shown in Supplementary Fig. 4 indicate that our spin-coated CH 3 NH 3 PbI 3- x Cl x perovskite thin films exhibit similar structural and optical properties as reported in literature [3] , [20] , [21] , [27] . Photovoltaic performance As described above, the UVO treatment of FTO substrates improves the quality of CH 3 NH 3 PbI 3- x Cl x films, and therefore is expected to improve cell performance. 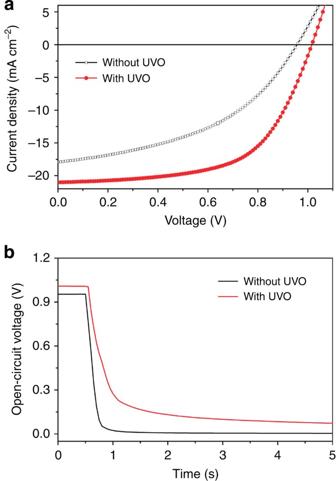Figure 3: Effects of UVO treatment. (a)J–Vcurves and (b)VOCdecay curves of two typical CH3NH3PbI3-xClx-based solar cells grown on FTO substrates with and without UVO treatment. Figure 3a shows the J – V curves of two typical CH 3 NH 3 PbI 3- x Cl x -based solar cells grown on FTO substrates with (solid red curve) and without (open black curve) UVO treatment. The cell grown on FTO substrate with UVO treatment exhibited a V OC of 1.02 V, a short-circuit current ( J SC ) of 21.02 mA cm −2 , a FF of 0.59 and a PCE of 12.72%. However, the cell fabricated with identical conditions but on a FTO substrate without UVO treatment showed a V OC of 0.96 V, a J SC of 17.93 mA cm −2 , a FF of 0.45 and a PCE of 7.67%. Both cells were measured with a reverse voltage scan. Therefore, the observed differences are not caused by measurement variations. The series resistances ( R S ) of the cells grown on FTO substrates with and without UVO treatment are 3.90 and 7.19 Ω cm 2 , respectively. The shunt resistance ( R sh ) of the cells grown on FTO substrates with and without UVO treatment are 900 and 360 Ω cm 2 , respectively. It is seen that the UVO treatment of FTO substrates improves the J SC , FF, V OC and PCE, reduces the R S and increases the R sh . This is consistent with the observation that UVO treatment of FTO substrates improves the smoothness and coverage of CH 3 NH 3 PbI 3- x Cl x films. The improved coverage should reduce the amount of direct contact between the FTO and the HTL, which should result in increased R sh and carrier lifetime, and therefore V OC . Furthermore, UVO treatment has also been widely reported to increase the work functions of metal oxides [28] , [29] , [30] , [31] . It is possibly through the reduction of the concentration of oxygen vacancy and therefore a downshift of Fermi level [31] . It has already been confirmed that UVO treatment has an effect on electrical and photovoltaic properties of metal oxides [28] , [29] . A reduced electron concentration of the FTO surface layer is expected to lower interfacial recombination and improve V OC . These are confirmed by the V OC decay measurements, which are related to the charge carrier recombination rate and the carrier lifetime [32] , [33] . The measured V OC decay curves of two representative perovskite solar cells grown on FTO substrates with and without UVO treatment are shown in Fig. 3b . The cell grown on FTO substrate with UVO treatment exhibited a longer V OC decay time than the cell grown on FTO substrate without UVO treatment. Figure 3: Effects of UVO treatment. ( a ) J – V curves and ( b ) V OC decay curves of two typical CH 3 NH 3 PbI 3- x Cl x -based solar cells grown on FTO substrates with and without UVO treatment. Full size image The thickness of the light-absorbing layer plays an important role in determining the performance of thin-film solar cells [34] . If the absorber layer is too thin, not enough light will be absorbed, which will lead to low current. If the absorber layer is too thick, the phtotogenerated carriers cannot be collected effectively because they must travel through the absorber layer and reach the carrier collecting layers before they recombine. We have investigated the effects of the CH 3 NH 3 PbI 3- x Cl x film thickness on the device performance. The measured J – V curves under reverse voltage scans are shown in Fig. 4 . Table 1 shows the photovoltaic parameters of perovskite solar cells with various absorber thicknesses grown on FTO substrates with UVO treatment. It is seen that both the V OC and J SC increase as the thickness of the CH 3 NH 3 PbI 3- x Cl x film increases. However, the FF first increases then decreases as the thickness of the CH 3 NH 3 PbI 3- x Cl x film increases. As a result, the PCE also first increases and then decreases as the thickness of the CH 3 NH 3 PbI 3- x Cl x film increases. The optimum thickness of the perovskite CH 3 NH 3 PbI 3- x Cl x film is ~500 nm. 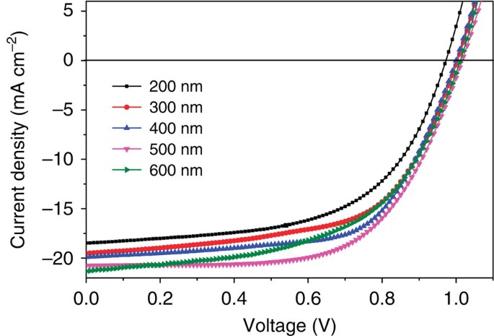Figure 4: Photocurrent density–voltage curves. MeasuredJ–Vcurves of CH3NH3PbI3-xClx-based solar cells with various absorber thicknesses. The thicknesses of the perovskite films were controlled by the spin rate. Figure 4: Photocurrent density–voltage curves. Measured J – V curves of CH 3 NH 3 PbI 3- x Cl x -based solar cells with various absorber thicknesses. The thicknesses of the perovskite films were controlled by the spin rate. Full size image Table 1 Photovoltaic parameters of the perovskite solar cells. Full size table It is noted that including Cl in the precursors is another key for realizing high V OC CH 3 NH 3 PbI 3- x Cl x -based solar cells grown directly on FTO substrates without any HBLs. CH 3 NH 3 PbI 3 -based solar cells grown directly on FTO substrates without any HBLs have exhibited extremely poor FFs and V OC ’s ( Supplementary Fig. 5 ). The dark J – V curve indicates a poor rectify behaviour, a common feature for cells with direct contacts between absorbers and electrodes. The poor V OC is expected because holes generated in CH 3 NH 3 PbI 3 will recombine with electrons from the FTO substrate. X-ray diffraction and SEM ( Supplementary Fig. 6 ) showed that CH 3 NH 3 PbI 3 thin films exhibited similar coverage and crystallinity as CH 3 NH 3 PbI 3- x Cl x thin films. The high V OC ’s seen in CH 3 NH 3 PbI 3- x Cl x -based solar cells should, therefore, not be due to Cl-enhanced film quality. A recent theoretical study has shown that Cl may segregate to and passivate TiO 2 /CH 3 NH 3 PbI 3- x Cl x interface, leading to enhanced carrier lifetime [35] . Passivation of interfaces at electron collecting layer and perovskite films has been found to improve the performance of perovskite solar cells [36] . To investigate the charge extraction process in CH 3 NH 3 PbI 3- x Cl x and CH 3 NH 3 PbI 3 films, we performed time correlated single-photon counting luminescence decays for the CH 3 NH 3 PbI 3- x Cl x and CH 3 NH 3 PbI 3 ( Supplementary Fig. 7 ). The PL quenching measurements are related to the electron–hole diffusion lengths and lifetimes [37] , [38] . As shown in Supplementary Fig. 7 , the CH 3 NH 3 PbI 3- x Cl x film has a longer charge–carrier lifetime than the CH 3 NH 3 PbI 3 film. Therefore, we speculate that the high V OC ’s achieved in CH 3 NH 3 PbI 3- x Cl x -based solar cells may be due to Cl-facilitated interface passivation. Similar effects have been observed in HCl-treated tin-doped indium oxide substrates used in organic photovoltaic cells [39] . Furthermore, as discussed earlier, UVO treatment to FTO substrates may also help reduce interface recombination. Cl in precursors has also been found to improve perovskite film quality such as coverage [40] , [41] . However, we did not observe significant difference on film coverage for CH 3 NH 3 PbI 3 and CH 3 NH 3 PbI 3- x Cl x films in our study. We have tried with great efforts to measure Cl concentration at FTO/CH 3 NH 3 PbI 3- x Cl x interfaces, but no noticeable Cl has been found. We suspect that the amount of Cl present at FTO/CH 3 NH 3 PbI 3- x Cl x interfaces could be below the detection limit of our instrument. Further investigations are needed to understand the effects of Cl. Junction properties The J – V curves of the best-performing CH 3 NH 3 PbI 3- x Cl x -based solar cell grown directly on a UVO-treated FTO substrate, under illumination and in the dark, are shown in Fig. 5a . This cell has achieved a maximum PCE of 14.14% with a V OC of 1.06 V, a J SC of 19.76 mA cm −2 and a FF of 0.67 under the reverse voltage scan with a scan rate of 0.1 V s −1 . It is well known that perovskite solar cells exhibit hysteresis effect, especially the cells with a planar structure [36] , [42] . We have observed similar hysteresis behaviours in our perovskite cells grown directly on FTO substrates, as shown in Supplementary Fig. 8 and Supplementary Table 1 . For the same device, the V OC , J SC , FF and PCE depend on both the voltage scan direction and rate. The V OC , J SC , FF and PCE are 1.04 V, 19.78 mA cm −2 , 0.65 and 13.35%, respectively, when measured under a reverse scan (from V OC to 0 V) with a scan rate of 0.1 V s −1 , whereas the V OC , J SC , FF and PCE are 0.96 V, 19.97 mA cm −2 , 0.52 and 10.04%, respectively, when measured under forward scan (from 0 V to V OC ) with the scan rate of 0.1 V s −1 . Clearly, with the same scan rate, the reverse scan resulted in higher V OC , FF and PCE than the forward scan. Furthermore, the higher scan rate resulted in a higher efficiency for the same scan direction. For example, under reverse scan, the 0.1 V s −1 scan rate showed a PCE of 13.35%, while the 0.01 V s −1 scan rate showed a PCE of 11.23%. Supplementary Fig. 9 and Supplementary Table 2 show the J – V curves of a representative HBL-free cell measured under forward and reverse voltage scans with five cycles. A stable average efficiency of 11.26% was achieved after the cell measured with five cycles. It has been demonstrated that hysteresis of perovskite solar cells can be reduced or even eliminated by special interface passivation [36] . Therefore, further work is needed to reduce or eliminate the hysteresis in our cells. 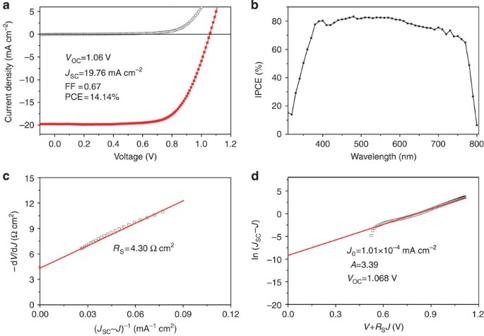Figure 5: Photovoltaic and junction performances. (a)J–Vcurves of the best-performing cell composed of UVO-treated FTO/500 nm CH3NH3PbI3-xClx/spiro-OMeTAD/Au under AM1.5 simulated irradiation (closed red squares) and in the dark (open black squares). (b) IPCE spectrum of the best-performing cell composed of UVO-treated FTO/500 nm CH3NH3PbI3-xClx/spiro-OMeTAD/Au. (c) The linear curve of the relationship of −dV/dJand (JSC−J)−1. (d) The plot of the relationship of ln(JSC−J) andV+RSJ. The junction properties are based on the best-performing cell. The red lines are best linear fits to the data. Figure 5b shows the incident photon-to-current conversion efficiency (IPCE) spectrum of this cell. The IPCE spectrum shows efficiencies of ~80% in the 400–750-nm wavelength range, which is consistent with the ultraviolet–visible absorbance of the perovskite CH 3 NH 3 PbI 3- x Cl x film. The dark current density–voltage curve of the solar cell based on the CH 3 NH 3 PbI 3- x Cl x film shows good rectification characteristics ( Fig. 5a ). Figure 5: Photovoltaic and junction performances. ( a ) J – V curves of the best-performing cell composed of UVO-treated FTO/500 nm CH 3 NH 3 PbI 3- x Cl x /spiro-OMeTAD/Au under AM1.5 simulated irradiation (closed red squares) and in the dark (open black squares). ( b ) IPCE spectrum of the best-performing cell composed of UVO-treated FTO/500 nm CH 3 NH 3 PbI 3- x Cl x /spiro-OMeTAD/Au. ( c ) The linear curve of the relationship of −d V /d J and ( J SC − J ) −1 . ( d ) The plot of the relationship of ln( J SC − J ) and V + R S J . The junction properties are based on the best-performing cell. The red lines are best linear fits to the data. Full size image Because the J – V curves show good rectification characteristics, the R S and V OC of the cell can be calculated according to the diode equation [14] : where T is the absolute temperature, K B is Boltzmann constant, A is ideality factor and J 0 is the reverse saturated current density [14] . The R S and V OC can be obtained from equations (1) and (3), respectively. Figure 5c shows a linear relationship between −d V /d J and ( J SC − J ) −1 . The value of R S is equal to the intercept on the y axis. The R S of the device without a conventional HBL is 4.30 Ω cm 2 . According to equation (2), J 0 is equal to the y intercept of the line in Fig. 5d . The values of J 0 and A are 1.01 × 10 −4 mA cm −2 and 3.39, respectively. According to equation (3), the calculated value of the V OC is 1.068 V; this calculated value is very close to the value obtained from the J – V measurement. Reproducibility and stability To check the reproducibility of the performance of the simple heterojunction perovskite solar cells, we fabricated and measured 56 separate devices. Supplementary Figure 10 shows the histograms of the photovoltaic parameters. The average values of V OC and J SC are 1.00 V and 20.08 mA cm −2 , respectively. Most of the devices show a PCE higher than 11%, revealing a high reproducibility. Supplementary Figure 11 shows the results of long-term stability tests of the devices without HBLs. The test was done by measuring the J – V curves of the devices after stored for a certain period of time. The tested devices were not encapsulated and were stored in atmosphere with humidity of 20% and at room temperature without light illumination. The values of FF and PCE first increased and then decreased. The values of V OC remained unchanged for a long period. The initial increase in cell performance may be attributed to oxygen-induced doping of spiro-OMeTAD, which has been reported in literature [43] , [44] . The PCE of the non-encapsulated perovskite solar cell was >70% of its initial value after 500 h ( Supplementary Fig. 11 ). The highest V OC achieved with our CH 3 NH 3 PbI 3- x Cl x -based perovskite solar cells grown directly on FTO substrates without any HBLs is 1.06 V. As the perovskite layers were deposited by the one-step spin-coat process, remnant PbI 2 layers acting as HBLs can be excluded. Such a high V OC is unexpected for a solar cell grown directly on a conductive electrode. As discussed above, including Cl and applying UVO treatment to FTO substrates are the key for achieving the high V OC ’s. To test if including a TiO 2 HBL would further significantly improve the V OC , we have incorporated a thin layer of TiO 2 on FTO substrates. 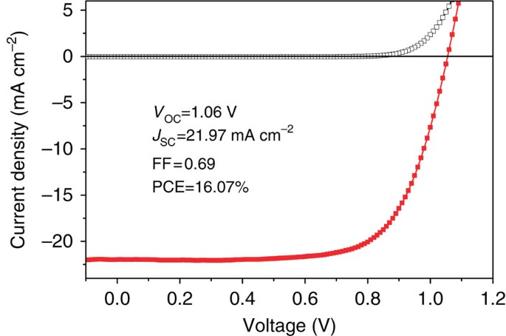Figure 6: Cell performance. J–Vcurves of a perovskite-based solar cell composed of FTO/60 nm TiO2/500 nm CH3NH3PbI3-xClx/spiro-OMeTAD/Au. Figure 6 shows the J – V curves (reverse scan) of the best-performing CH 3 NH 3 PbI 3- x Cl x -based solar cell with a 60-nm-thick undoped TiO 2 layer. The obtained V OC is ~1.06 V. It is seen that the cell efficiency has been improved. Surprisingly, however, there was no improvement on the V OC . The efficiency improvement was due to the enhancements of FF and J SC . As speculated, Cl may diffuse to and passivate FTO/CH 3 NH 3 PbI 3- x Cl x interfaces, and lead to the observed high V OC ’s for CH 3 NH 3 PbI 3- x Cl x -based perovskite solar cells grown directly on FTO substrates without HBLs. The passivation seems to be as effective as the TiO 2 HBL. Therefore, our results suggest that TiO 2 may not be the ultimate HBL material for achieving high-efficiency lead halide perovskite solar cells. We anticipate that other oxide-based HBLs may also be able to produce high-efficiency lead halide perovskite solar cells and should be explored. While this paper was under review, a relevant paper was published [45] . It was suggested that the remnant PbI 2 layer, an unavoidable residual layer for the two-step process, at FTO/CH 3 NH 3 PbI 3 interface could act as a HBL. Figure 6: Cell performance. J – V curves of a perovskite-based solar cell composed of FTO/60 nm TiO 2 /500 nm CH 3 NH 3 PbI 3- x Cl x /spiro-OMeTAD/Au. Full size image In summary, we have demonstrated high V OC efficient planar CH 3 NH 3 PbI 3- x Cl x -based thin-film solar cells grown directly on FTO glass substrates without any HBLs. The best-performing perovskite solar cell has achieved a PCE of 14.14% and a high V OC of 1.06 V. This V OC is as high as our best reference cell using a TiO 2 HBL (PCE=16.07%, V OC =1.06 V). We have shown that UVO treatment of FTO substrates and including Cl in precursors are two key factors that ensure the high V OC for lead halide perovskite solar cells grown directly on FTO substrates without HBLs. While the actual mechanism deserves more careful study, our results strongly suggest that TiO 2 may not be the ultimate HBLs for achieving high-efficiency lead halide perovskite solar cells. Our results also provide insights on how to improve the performance of lead halide perovskite solar cells using other metal oxides. Solar cell fabrication The perovskite CH 3 NH 3 PbI 3 and CH 3 NH 3 PbI 3- x Cl x films were synthesized by the one-step process as reported in literature [6] , [46] , [47] . First, 19.8 ml (0.15 mol) hydroiodic acid (Sigma-Aldrich, 57 wt.% in water, 99.99%) and 18.7 ml (0.15 mol) methylamine (Sigma-Aldrich, 33 wt.% in absolute ethanol) at a 1:1 equimolar ratio were stirred in an ice bath for 2 h. The precipitate was collected by evaporating at 50 °C for 2 h. Finally, a white powder was received by washing with diethyl ether and ethanol three times and then drying at 100 °C in a vacuum oven for 24 h. A precursor solution of CH 3 NH 3 PbI 3- x Cl x was composed of CH 3 NH 3 I and PbCl 2 (Aladdin reagent, 99.99%) with a molar ratio of 3:1. The precursor solution of CH 3 NH 3 PbI 3 was composed of CH 3 NH 3 I and PbI 2 (Aladdin reagent, 99.99%) with a molar ratio of 1:1. The solvent of the two precursor solutions was anhydrous dimethylformamide (Sinopharm Chemical Reagent Co., Ltd). The solutions were stirred at room temperature for 24 h. TiO 2 film coated on FTO substrate was prepared by a spin-coating method and was sintered at 500 °C for 30 min (refs 48 , 49 ). The perovskite CH 3 NH 3 PbI 3 and CH 3 NH 3 PbI 3- x Cl x films coated on FTO glasses (Asahi Glass, 14 Ohm per square) were prepared by a spin-coating method. The thicknesses of the CH 3 NH 3 PbI 3- x Cl x films were controlled by the spin rate with a same solution. The FTO glasses were treated with UVO for 30 min. Before spin coating, the precursor solutions and the substrates were preheated at 60 °C for 15 min. The perovskite CH 3 NH 3 PbI 3- x Cl x and CH 3 NH 3 PbI 3 films were heated at 100 °C in a vacuum oven for 45 and 15 min, respectively. The hole-transporting material was composed of 68 mM spiro-OMeTAD (Shenzhen Feiming Science and Technology Co., Ltd, 99.0%), 26 mM Li-TFSI (Aladdin reagent) and 55 mM TBP (Aladdin reagent). The solvent was a mixed solution of acetonitrile and chlorobenzene with a volume ratio of 1:10. It was stirred at room temperature for 24 h and then was used to coat the perovskite films by a spin-coating method at a speed of 2,000 r.p.m. for 30 s. Device fabrication was completed by deposition of a thin gold electrode on the HTL. The active areas of the devices were controlled by a shadow mask in the thermal evaporator. Characterization The morphologies of perovskite solar cells were observed by a high-resolution field emission SEM (JSM 6700F). The absorption and transmission spectra of the perovskite CH 3 NH 3 PbI 3- x Cl x film on FTO was measured by an ultraviolet–visible spectrophotometer (CARY5000, Varian, Australia) in the 400–800-nm wavelength range at room temperature. Hall measurements were conducted via a LakeShore 7704 Hall Measurement System. PL spectrum was obtained with a 532-nm laser, as the excitation source, pulsed at a frequency of 9.743 MHz. The perovskite solar cells were stored in ambient air for a short period of time and then measured under a 100 mW cm −2 (AM1.5 simulated irradiation) illumination with a standard ABET Sun 2000 Solar Simulator. The light intensity was calibrated by a standard silicon solar cell. The cell size was 2 cm × 2 cm. The active area was 0.09 cm 2 , which was defined by the area of the Au electrode. The J – V characteristics were measured by a CHI660D electrochemical workstation (ShangHai, China). The IPCE spectrum was measured by a Quantum Efficiency/IPCE system (PV Measurements Inc.) in the 320–800-nm wavelength range at room temperature. All the efficiencies were taken from the initial measurement, except for the test of the stability. How to cite this article: Ke W. et al . Efficient hole-blocking layer-free planar halide perovskite thin-film solar cells. Nat. Commun. 6:6700 doi: 10.1038/ncomms7700 (2015).